A causal role of the right inferior frontal cortex in implementing strategies for multi-component behaviour Everyday activities, such as, for example, driving a car or preparing a meal, require the hierarchical organization and processing of several individual actions. Currently, the neural mechanisms underlying the control of action sequences are not well understood. Here, the authors demonstrate that the right inferior frontal gyrus (rIFG) plays a key role in implementing the strategy used to cascade different actions. Continuous theta burst stimulation (TBS) applied to the rIFG results in a less efficient action cascading strategy, whereas intermittent TBS results in a more efficient strategy, compared with a shamTBS control condition. These effects are confirmed in electrophysiological data showing that activity differences in the rIFG are related to alterations in response selection processes. Overall, these results suggest that the neural dynamics of the rIFG determine the strategy used during some forms of everyday multi-component behaviour. Steering, braking, switching gears and tuning the radio of a car require complex coordination of actions. Such coordination requires the organization of individual actions into a hierarchical structure that can be flexibly interrupted and altered to achieve a goal whenever necessary. A number of previous studies have demonstrated that people apply different strategies when coordinating complex motor plans [1] , [2] , [3] in situations requiring a chaining of different actions to achieve a goal; however, the neuronal mechanisms underlying the strategy that links individual actions in multi-component behaviour have remained elusive. Studies from the field of cognitive psychology suggest rapid and efficient unfolding of behaviour can be accomplished using a serial processing strategy in which one task goal is activated after the previous goal has been carried out. However, an alternative strategy in which different task goals are activated with some temporal overlap (that is, parallel processing) hampers the efficient unfolding of multi-component behaviour, possibly because different actions interfere with each other and overstrain response selection capacities [1] , [2] , [3] , [4] . Several lines of evidence suggest that the right inferior frontal gyrus (rIFG) is important for the hierarchical organization and processing of actions during multi-component behaviour [5] , [6] , [7] . The rIFG has been suggested to link different actions to enable a smooth unfolding of multi-component behaviour [8] , and is therefore critically involved in organizing the individual components of action sequences [9] , [10] . Given that the rIFG plays a key role in multi-component behaviour [5] , it may also determine the strategy used during multi-component behaviour. Thus, it should be possible to manipulate processing strategies and therefore the efficacy of multi-component behaviour by altering the neuronal processes within the rIFG. Continuous theta burst stimulation (cTBS) and intermittent TBS (iTBS) have been shown to induce opposing effects in neural circuits [11] , [12] , as they transiently inhibit and facilitate neural dynamics, respectively [11] , [12] , [13] . In three sessions, we applied cTBS, iTBS or shamTBS to the rIFG of healthy adult subjects. We hypothesized that the bi-direction effects of TBS on neural dynamics would result in bi-directional shifts in the strategy used during multi-component behaviour. To examine multi-component behaviour, we applied a stop–change paradigm [1] , [3] ( Fig. 1 ) in which subjects were required to make rapid responses to stimuli presented on a screen. Occasionally, a reaction was interrupted following delivery of a STOP stimulus, and an alternative response had to be executed upon the presentation of an auditory CHANGE stimulus. The CHANGE stimulus was presented either simultaneously with the STOP stimulus at a stop–change delay (SCD) of 0 ms or following the STOP stimulus at an SCD of 300 ms. For simultaneous STOP and CHANGE signals (SCD=0 ms), subjects could process the two actions either serially or in parallel; at an SCD of 300 ms, it was only possible to process the two actions in a step-by-step (that is, serial) manner [3] . As parallel strategies for individual action activation are related to inefficient unfolding behaviour [1] , [3] , [4] , they typically result in longer reaction times (RTs) on the CHANGE signal (RT2). Using these SCD manipulations and applying mathematical constraints to the RT2 data allows inferences regarding the underlying processing strategy [3] . In the present study, we examined to what extent the neural dynamics in the rIFG, as modulated via iTBS or cTBS, are related to the inferred strategy and efficiency of multi-component behaviour. Moreover, by recorded event-related potentials (ERPs), we were able to identify associated alterations in cognitive processes on the attentional and response selection levels, both of which may contribute to shifts in multi-component processing strategies [1] , [14] , [15] . cTBS applied to the rIFG results in a less efficient action cascading strategy, whereas iTBS results in a more efficient strategy, compared with a shamTBS control condition. These effects are confirmed in electrophysiological data, showing that activity differences in the rIFG are related to alterations in response selection processes. Overall, these results suggest that the neural dynamics of the rIFG determine the strategy used during some forms of everyday multi-component behaviour. 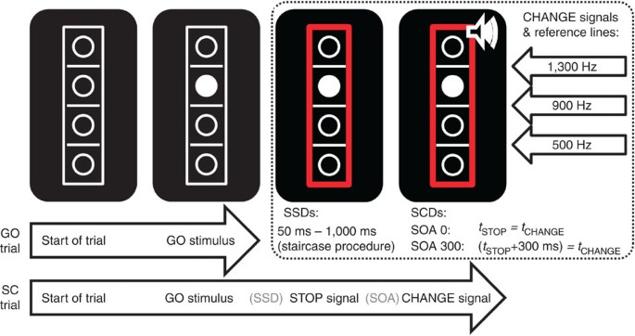Figure 1: Schematic illustration of the stop–change paradigm. GO trials end after the first response to the GO stimulus (bold). In contrast, SC trials end after the first response to the CHANGE signal (bold). SC trials are constituted by stopping of the GO response upon presentation of the STOP signal. The stop-signal delay (SSD) between the onset of the GO stimulus and the STOP signal was adjusted using a staircase procedure described in the Methods section. After stopping, an alternative response on the CHANGE stimulus is executed. The stimulus onset asynchrony (SOA) between the onset of the STOP and CHANGE stimuli was set to either 0 or 300 ms. As indicated in the upper right corner, the three CHANGE stimuli were associated with one of the three reference lines (white horizontal lines in the rectangle containing the dots). Figure 1: Schematic illustration of the stop–change paradigm. GO trials end after the first response to the GO stimulus (bold). In contrast, SC trials end after the first response to the CHANGE signal (bold). SC trials are constituted by stopping of the GO response upon presentation of the STOP signal. The stop-signal delay (SSD) between the onset of the GO stimulus and the STOP signal was adjusted using a staircase procedure described in the Methods section. After stopping, an alternative response on the CHANGE stimulus is executed. The stimulus onset asynchrony (SOA) between the onset of the STOP and CHANGE stimuli was set to either 0 or 300 ms. As indicated in the upper right corner, the three CHANGE stimuli were associated with one of the three reference lines (white horizontal lines in the rectangle containing the dots). Full size image TBS of rIFG influences the action strategy The location of the stimulated area in the rIFG is shown in Fig. 2a . The behavioural data show that on uninterrupted trials (gene ontology (GO) trials), RTs did not differ across the three TBS conditions. In addition, the stop-signal RT (SSRT) did not differ across TBS conditions in univariate analyses of variance (ANOVAs) (all F<1.2; P >0.4). The SSRT is the average ‘go’ response time minus the average ‘stop’ signal presentation time for successful stopping. Note that the SSRT is measured in all stop–change trials and is distinct from the RT to the change stimulus (RT2), which is plotted in Fig. 2b . The three TBS protocols resulted in differential modulation of RT2 on stop–change trials. Moreover, RT2 also varied across the two SCD conditions. These results were confirmed by a significant interaction effect of ‘SCD × TBS protocol’ in a mixed-effects ANOVA (F(2,34)=22.19; P <0.001; η 2 =0.557), as shown in Fig. 2b . 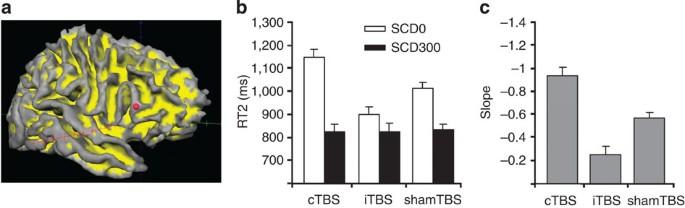Figure 2: Behavioural results and TBS target zone. (a) Localization of the stimulation area within the rIFG. The red dot denotes the point of stimulation in the rIFG. (b) Mean reaction time data (based on∼130 repetitions for each SCD interval) (±s.e.m.) (n=18 subjects) on the CHANGE stimuli (that is, RT2) for the SCD0 and SCD300 conditions for the different experimental sessions using shamTBS, iTBS or cTBS (left part of the figure). (c) Mean slope of the SCD-RT2 function (±s.e.m.) for the different experimental sessions (shamTBS, iTBS or cTBS). Figure 2: Behavioural results and TBS target zone. ( a ) Localization of the stimulation area within the rIFG. The red dot denotes the point of stimulation in the rIFG. ( b ) Mean reaction time data (based on ∼ 130 repetitions for each SCD interval) (±s.e.m.) ( n =18 subjects) on the CHANGE stimuli (that is, RT2) for the SCD0 and SCD300 conditions for the different experimental sessions using shamTBS, iTBS or cTBS (left part of the figure). ( c ) Mean slope of the SCD-RT2 function (±s.e.m.) for the different experimental sessions (shamTBS, iTBS or cTBS). Full size image In SCD300 trials, where the change signal followed the stop signal with a delay of 300 ms, RT2 was similar across TBS protocols ( P >0.6). However, in the more difficult SCD0 condition, in which STOP and CHANGE stimuli were presented simultaneously, there were significant differences in RT2s across TBS protocols ( P <0.001, Bonferroni corrected). Compared with the shamTBS condition (average RT2=1,013 ms±27), the cTBS protocol produced a slowing of RT2s (1,108 ms±34), whereas the iTBS protocol increased the speed of RT2s (898 ms±35). The slope of the SCD-RT2 functions provides insights into the mode of action cascading [1] , [3] induced by the different TBS protocols. Here, we found that the slope differed across TBS protocols (F(2,34)=22.19; P <0.001; η 2 =0.566; see Fig. 2c ). The slope was steepest in the cTBS session (−0.94±0.05) and flattest in the iTBS session (−0.25±0.07). Pairwise comparisons revealed that all conditions differed from each other ( P <0.001), suggesting a more parallel strategy of goal activation during cTBS and a more serial strategy of goal activation during iTBS. During shamTBS, the slope fell midway between that measured in the cTBS and iTBS sessions (−0.61±0.08; P <0.001), and was significantly different from both ( P <0.10). These results were not influenced by the presence of the TBS equipment, as the shamTBS slope was comparable to what is usually observed in healthy subjects not undergoing TBS [1] , [3] , [4] . No effect of other multiple-demand system regions To test the specificity of the effects obtained for the rIFG, we examined TBS effects in two other target zones in the frontal and inferior parietal cortex in separate behavioural experiments with n =10 subjects each. The target zones and the results obtained are shown in Fig. 3 . The results obtained for the target zone in the right middle frontal gyrus [ x , y , z =41, 23, 29] are shown in Fig. 3a . The reason for choosing these coordinates was that it is located adjacent to the rIFG and is also considered as a part of the multiple-demand system [5] . The RTs on GO trials did not differ between TBS conditions as shown in univariate ANOVAs (all F<0.7; P >0.7; not shown in the figure). This parallels the findings obtained in the main experiment. The analysis of the RT2 data in CHANGE stimuli in mixed-effects ANOVAs showed that there was a main effect of ‘SCD interval’ (F(1,9)=93.59; P <0.001; η 2 =0.912). However, no interaction of the ‘SCD × TBS protocol’ (F(2,18)=0.02; P >0.9) and no main effect of the ‘TBS protocol’ (F(2,18)=0.27; P >0.7) were evident. Consequently, data analysis showed that the slope of the SCD-RT2 function did not differ between the shamTBS, iTBS and cTBS conditions (F(2,18)=0.02; P >0.9). This shows that TBS in this MFG control region did not modulate the processing strategy and hence the efficiency of action cascading, as it was the case for the rIFG target region in the main experiment. To further confirm this dissociation, we compared the slope of the SCD-RT2 function from this control experimental group with the behavioural data from the group undergoing stimulation of the rIFG. There were no group differences between the shamTBS conditions ( P >0.8), but between the iTBS and cTBS conditions of the main and control experiments: in the iTBS condition, the slope was smaller in the main experiment (rIFG target region) than in this control experiment using an MFG area ( P <0.001). In the cTBS condition, the slope was larger in the main experiment (rIFG target region) than in this control experiment ( P <0.001). This underlines that the modulation of the rIFG has an effect on the strategy and efficiency of action cascading while the target region in the right MFG does not. 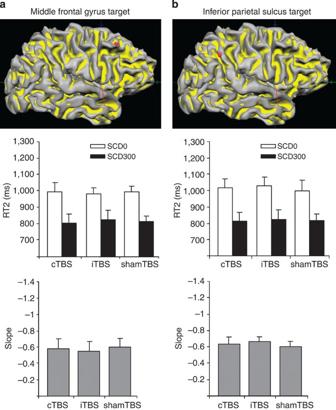Figure 3: Behavioural data from the experiments on two cortical control regions. (a) Results from the control experiment with the rMFG as the control region (n=10). (b) Results from the control experiment with the rIPS as the control region (n=10). On the top, the localization of the stimulation area within is shown. The red dot denotes the point of stimulation in the rMFG. In the middle the RT2 data (mean±s.e.m.) in the SCD0 and SCD300 are shown and at the bottom the slope of the SCD-RT2 function is shown (mean±s.e.m.). Figure 3: Behavioural data from the experiments on two cortical control regions. ( a ) Results from the control experiment with the rMFG as the control region ( n =10). ( b ) Results from the control experiment with the rIPS as the control region ( n =10). On the top, the localization of the stimulation area within is shown. The red dot denotes the point of stimulation in the rMFG. In the middle the RT2 data (mean±s.e.m.) in the SCD0 and SCD300 are shown and at the bottom the slope of the SCD-RT2 function is shown (mean±s.e.m.). Full size image An area in in the right inferior parietal sulcus (rIPS) was chosen as another target region [ x , y , z =37, −56, 41] because, like the right middle frontal gyrus, it is also part of the multiple-demand system [5] and is furthermore important for perceptual and attentional selection processes [16] , [17] . The results are shown in Fig. 3b . The RT on GO trials (not shown in the figure) did not differ between TBS conditions (all F<0.8; P >0.7). The RT data on the CHANGE stimuli (that is, RT2) showed a main effect of ‘SCD interval’ (F(1,9)=12.21; P =0.007; η 2 =0.576), but no interaction of the ‘SCD × TBS protocol’ (F(2,18)=0.08; P >0.9) and no main effect of the ‘TBS protocol’ (F(2,18)=0.03; P >0.9). There were hence no differences in the slope of the SCD-RT2 function between the shamTBS, iTBS and cTBS conditions (F(2,18)=0.08; P >0.9). As the rIFG group, this group was compared with the main experiment group where an area in the rIFG was stimulated. The slope of the SCD-RT2 function in the rIPS group differed from the iTBS and cTBS conditions of the main experiment targeting an area in the rIFG ( P <0.001). Again, this supports the specificity of the results obtained using the rIFG as target region for iTBS and cTBS. In sum, both control experiments (iIFG and rIPS) underline the specificity of the results obtained for TBS in the rIFG in the main experiment. Furthermore, the finding that none of the experimental groups showed TBS-induced RT differences in GO trials (all F<1.1; P >0.5) underlines that TBS specifically modulates stop–change processes. Evoked P3 amplitudes consistent with behaviour ERPs provide insights into the nature of the cognitive processes that are modulated. Perceptual and attentional mechanisms underlying visual STOP signal and auditory CHANGE signal processes are reflected by the P1 and N1 ERPs [18] , which were not differentially modulated by the SCD or TBS protocol (all F<1.2; P >0.4; see Fig. 4 ). 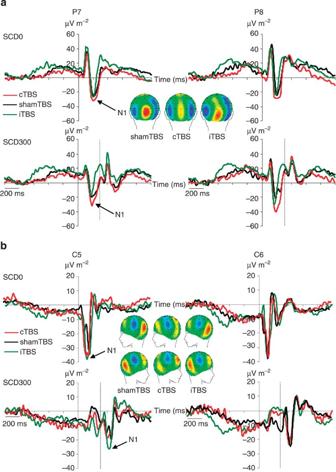Figure 4: Event-related potentials (P1 and N1). (a) Visual event-related current source densities (visual P1 and N1) at electrodes P7 and P8 (located at the back of the head) locked to the stop-stimulus presentation (that is, time point 0) for the different experimental sessions (shamTBS, iTBS and cTBS) in the SCD0 condition (top) and SCD300 condition (bottom); also shown are scalp topography maps (n=18). (b) Auditory event-related current source densities (P1 and N1) at electrodes C5 and C6 (located at the left and right side of the head). In the SCD300 condition, the dashed vertical line denotes the delivery of the CHANGE stimulus. Figure 4: Event-related potentials (P1 and N1). ( a ) Visual event-related current source densities (visual P1 and N1) at electrodes P7 and P8 (located at the back of the head) locked to the stop-stimulus presentation (that is, time point 0) for the different experimental sessions (shamTBS, iTBS and cTBS) in the SCD0 condition (top) and SCD300 condition (bottom); also shown are scalp topography maps ( n =18). ( b ) Auditory event-related current source densities (P1 and N1) at electrodes C5 and C6 (located at the left and right side of the head). In the SCD300 condition, the dashed vertical line denotes the delivery of the CHANGE stimulus. Full size image However, the P3 ERP, which has previously been shown to predict performance in this task [1] , [4] , showed an ‘SCD × TBS protocol’ interaction effect (F(2,34)=41.82; P <0.001; η 2 =0.71; see Fig. 5a ). Bonferroni-corrected post hoc tests showed that the TBS protocol did not influence the P3 amplitude in the SCD300 condition ( P >0.6), but it did in the SCD0 condition ( P <0.001). The pattern of the P3 electrophysiological data is therefore in line with the behavioural data. The P3 was larger in the cTBS session (57.21 μV m −2 ±4.6) and smaller in the iTBS session (18.86 μV m −2 ±2.8) as compared with that observed in the shamTBS session (40.4 μV m −2 ±2.9; P <0.001). Two separate standardized low-resolution brain electromagnetic tomography (sLORETA) source analyses [19] contrasting the cTBS and iTBS sessions against the shamTBS session in the SCD0 condition (cTBS>shamTBS and iTBS<shamTBS) confirmed that the differences between the conditions were due to activity differences in the rIFG (see Fig. 5b ). Correlation analyses indicated that the individual TMS-induced action selection mode differences as quantified on the behavioural level (that is, more serial in the iTBS session and more parallel in the cTBS session) were linearly correlated with differences in the electrophysiological data between the iTBS and shamTBS conditions ( r =0.755; P <0.001; R 2 =0.56), as well as the cTBS and shamTBS conditions ( r =0.684; P =0.001; R 2 =0.46; see Fig. 5c ). In Fig. 5c , all individual P3 amplitude and RT values obtained in the SCD0 condition of the shamTBS session were set to 0. 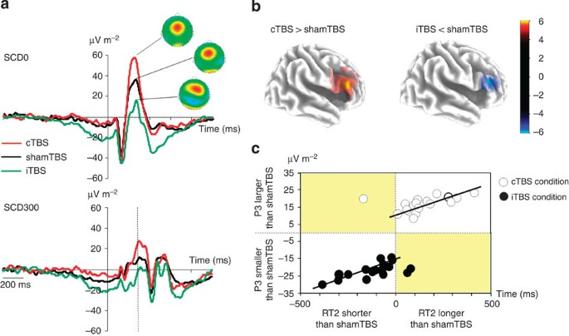Figure 5: Event-related potentials (P3). (a) P3 event-related current source densities at electrode Cz locked to the STOP-stimulus presentation (that is, time point 0) for the different experimental sessions (shamTBS, iTBS and cTBS) in the SCD0 condition (top) and SCD300 condition (bottom). Note that the scaling of the scalp topography plots is different for each TBS condition. Warm colours signal positivity. In the SCD300 condition, the dashed vertical line denotes the delivery of the change stimulus (n=18). (b) Plots showing the results of the sLORETA analysis comparing the iTBS and cTBS against the shamTBS condition. In both contrasts, activation differences in the rIFG are shown. The colour bar denotest-values showing the degree of activation differences as estimated using sLORETA. (c) Scatterplot denoting the correlations (Pearson correlations) between the two measures (behavioural/RT2s on thexaxis and neurophysiological/P3 amplitudes on theyaxis), which differed between iTBS and shamTBS (r=0.755;P<0.001;R2=0.56), as well as cTBS and shamTBS in the SCD0 condition (r=0.684;P=0.001;R2=0.46). For each participant, the values obtained in the shamTBS condition were set to be zero for both measures on both axes (see dotted lines in the middle of each axis). As can be seen, there was a positive correlation between RT2s and P3 amplitude: although iTBS improved (shortened) RT2s and reduced the P3 amplitude, cTBS worsened behavioural performance (prolonged RT2s) and increased P3 amplitudes. As can be seen in the yellow quadrants, only three subjects deviated from the expected outcome modulation. Figure 5c shows that, relative to this, the cTBS produced increases in P3 amplitude accompanied by longer RT2s, whereas the iTBS condition produced resulted in reductions in P3 amplitude accompanied by smaller RT2s. Therefore, both TBS manipulations are in line with the positive correlation between P3 amplitude and RT2s reported previously [1] , [4] . These results suggest that changes observed at the behavioural level are predictable from electrophysiological data and vice versa. As observed in the yellow quadrants of Fig. 5c , only one subject in the cTBS condition and two subjects in the iTBS condition deviated from the general pattern of TBS-induced RT2 modulation exhibited by the vast majority of subjects, demonstrating that the TBS-induced modulations were reliable even at the level of single subjects. Figure 5: Event-related potentials (P3). ( a ) P3 event-related current source densities at electrode Cz locked to the STOP-stimulus presentation (that is, time point 0) for the different experimental sessions (shamTBS, iTBS and cTBS) in the SCD0 condition (top) and SCD300 condition (bottom). Note that the scaling of the scalp topography plots is different for each TBS condition. Warm colours signal positivity. In the SCD300 condition, the dashed vertical line denotes the delivery of the change stimulus ( n =18). ( b ) Plots showing the results of the sLORETA analysis comparing the iTBS and cTBS against the shamTBS condition. In both contrasts, activation differences in the rIFG are shown. The colour bar denotes t -values showing the degree of activation differences as estimated using sLORETA. ( c ) Scatterplot denoting the correlations (Pearson correlations) between the two measures (behavioural/RT2s on the x axis and neurophysiological/P3 amplitudes on the y axis), which differed between iTBS and shamTBS ( r =0.755; P <0.001; R 2 =0.56), as well as cTBS and shamTBS in the SCD0 condition ( r =0.684; P =0.001; R 2 =0.46). For each participant, the values obtained in the shamTBS condition were set to be zero for both measures on both axes (see dotted lines in the middle of each axis). As can be seen, there was a positive correlation between RT2s and P3 amplitude: although iTBS improved (shortened) RT2s and reduced the P3 amplitude, cTBS worsened behavioural performance (prolonged RT2s) and increased P3 amplitudes. As can be seen in the yellow quadrants, only three subjects deviated from the expected outcome modulation. Full size image Validation of the shamTBS procedure For the shamTBS condition used in the main experiment and the control experiments outlined above, a standard procedure was used in which the coil was tilted away from the scalp in a 90° angle and a rubber spacer was placed between the subject’s head and the coil ( Fig. 6a ). To confirm whether the shamTBS as used in the main and control experiments is a valid control condition, we investigated whether it evokes functional changes as compared with a no-TBS baseline condition. For this purpose, we compared the behavioural and neurophysiological data obtained in the shamTBS condition of the main experiment group with a group ( n =15) performing the stop–change task without any TBS intervention (that is, a no-sham no-TBS control condition). Behavioural and neurophysiologic results are shown in Fig. 6b,c . As can be seen, there were no differences between participants undergoing shamTBS in the main experiment and participants in the no-sham no-TBS control group as tested using univariate and mixed-effects ANOVAs (all F<0.9; P >0.5). The same can be observed for the neurophysiological data (P3 ERP) ( Fig. 6b ) obtained in the SCD0 and SCD300 conditions. All in all, there were no differences between participants undergoing shamTBS (taken from the main experiment) and participants in the no-sham no-TBS control group (orange line in the ERPs) (all F<0.4; P >0.7). This demonstrates that the sham procedure used does not evoke functional changes as compared with a no-TBS baseline. 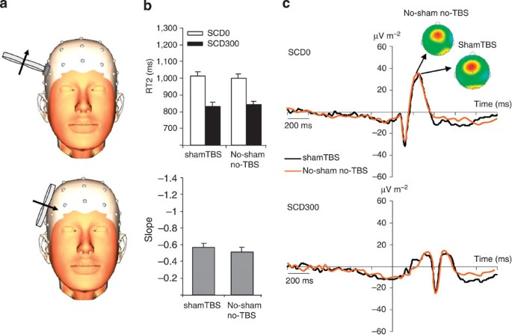Figure 6: Results for the shamTBS validation procedure. (a) Schematic illustration of the TMS coil orientation on the sham TBS (top) and iTBS/cTBS condition (bottom). The black arrow denotes the direction of the magnetic field. In the shamTBS condition, the TMS coil is tilted away by 90 degrees relative to the iTBS and cTBS conditions. Therefore, the magnetic field does not affect the cortex. To ensure that residual magnetic influences from the outer parts of the coil cannot have an effect, a piece of rubber was placed between the TMS coil and the head (left part of the picture). The heads show the used electroencephalogram electrode grid. The head was taken from the BrainVision Analyzer II software package. (b) Reaction time data (mean±s.e.m.) based on∼130 repetitions for each SCD interval (top) and the slope of the SCD-RT2 function (bottom) (n=15). (c) Event-related potential (P3) data in the SCD0 and SCD300 for the no-sham no-TBS group and the shamTBS group. Warm colours signal positivity in the scalp topography plots. Figure 6: Results for the shamTBS validation procedure. ( a ) Schematic illustration of the TMS coil orientation on the sham TBS (top) and iTBS/cTBS condition (bottom). The black arrow denotes the direction of the magnetic field. In the shamTBS condition, the TMS coil is tilted away by 90 degrees relative to the iTBS and cTBS conditions. Therefore, the magnetic field does not affect the cortex. To ensure that residual magnetic influences from the outer parts of the coil cannot have an effect, a piece of rubber was placed between the TMS coil and the head (left part of the picture). The heads show the used electroencephalogram electrode grid. The head was taken from the BrainVision Analyzer II software package. ( b ) Reaction time data (mean±s.e.m.) based on ∼ 130 repetitions for each SCD interval (top) and the slope of the SCD-RT2 function (bottom) ( n =15). ( c ) Event-related potential (P3) data in the SCD0 and SCD300 for the no-sham no-TBS group and the shamTBS group. Warm colours signal positivity in the scalp topography plots. Full size image In the current study, we examined the role of the rIFG in determining the strategy used to chain different actions during multi-component behaviour. Previous studies showed that the (r)IFG is important for the hierarchical organization and processing of actions during multi-component behaviour [5] , [6] , [7] , [8] , [9] , [10] ; however, the neural mechanisms mediating the implementation of a particular processing strategy have remained elusive. Understanding these mechanisms is important because the processing strategy ultimately determines the efficacy of multi-component behaviour. Our results demonstrate that it is possible to bi-directionally shift the processing strategy so that action cascading is either more or less effective. In the SCD0 condition, in which participants had to choose how to process two simultaneously triggered actions (stopping an ongoing response and changing to another response), iTBS of the rIFG induced a more efficient strategy of task goal activation, while cTBS of the rIFG induced a less efficient strategy of task goal activation compared with shamTBS. Although cTBS is thought to predominantly induce transient suppression and iTBS facilitation of neural circuits [11] , [12] , the effects of iTBS on the prefrontal cortex are less substantiated than the effects of cTBS [11] , [20] . Our data therefore suggest that the facilitation of neural processing in the rIFG promotes selection of a strategy that hierarchically structures actions, which in turn leads to a more efficient unfolding of multi-component behaviour, as reflected by the RT data. Likewise, the suppression of neural processing in the rIFG tended to impede the establishment of a strategy for hierarchically structuring actions, particularly in situations in which subjects were able to ‘choose’ between different response selection strategies (that is, SCD0). Overall, we found that external TBS modulation of the rIFG strongly modifies the strategy that subjects select to cope with situations requiring multi-component behaviour. The control experiments show that these effects are specific to the rIFG, as modulation of areas in the middle frontal gyrus and the inferior parietal cortex did not result in strategy alternations. Despite the fact that the (r)IFG is only one of many brain structures in a broad network involved in multi-component behaviour [5] , the current results suggest that the rIFG plays a critical role because the stimulation of an area alone was sufficient to influence the selected processing strategy and hence the efficacy of multi-component behaviour. In line with this interpretation, the stimulation of an inferior parietal target zone as well as another target region in the frontal cortex (both parts of the multiple-demand system [5] ) did not change the strategy used during action cascading. While these results underscore the previously established importance of the IFG in the processing of hierarchical sequential domains [6] , [7] , [8] , [9] , they broaden the role attributed to the IFG by showing that the IFG also determines the strategy and efficacy of human multi-component behaviour. The ERP data indicate that the rIFG determines the applied strategy by selectively modulating processes at the response selection level, leaving perceptual and attentional selection processes unaffected. This was evidenced by the fact that P3 was modulated by TBS while the visual and auditory P1 and N1 (reflecting attentional selection processes) were unaffected [1] , [21] . In this context, a larger P3 amplitude was associated with a less efficient processing strategy [1] , [21] . In the stop–change paradigm used in the present experiments, P3 likely reflects behavioural inhibition and change processes. This interpretation seems particularly poignant for the SCD0 condition, in which TBS protocols showed differential effects. As discussed in previous studies [21] , the more that participants attempt to simultaneously process the ‘stop-goal’ and the ‘change-goal’, the stronger the interference between these goals at a strategic response selection bottleneck [3] . Inhibitory control processes that manage the stopping of a response are likely to be intensified as a result of stronger interference. Such amplifications of response inhibition efforts have been shown to correlate with higher P3 amplitudes [22] . Changes in the efficacy of multi-component behaviour (as shown by the RT data) are direct consequences of the changes induced in neural processes related to the selection of responses. The ventral and dorsal part of the rIFG are differentially involved in the updating of action plans and attentional functions, respectively [14] . Verbruggen et al. [14] showed that stimulating coordinates in the rIFG similar to those in our study led to changes in response selection but not attentional selection processes. This is the likely reason explaining why changes in strategy are related to changes in response selection processes and not attentional selection processes. Furthermore, we did not observe changes in the SSRT (an indicator of inhibition/stopping processes) despite the fact that regions in the rIFG similar to those stimulated in current study have previously been demonstrated to modulate SSRTs [14] , [23] , [24] , [25] , [26] . However, it has previously been shown that the stopping and changing processes for the current task may be represented as a single task goal [3] . Therefore, the present study is therefore not completely comparable to the classical stop signal task. In addition, in our other studies using this task, the SSRT did not change when different modes of task goal processing were used [1] , [4] . These results are consistent with recent studies suggesting that the rIFG is unlikely to reflect a specific module for inhibitory demands [27] but is instead also part of other cognitive domains. In summary, the present study highlights the possibility that directly manipulating neural processing in the rIFG can lead to bi-directional shifts in action coordination strategies and therefore influence the efficacy of human multi-component behaviour. The rIFG appears to determine the strategy applied when presented with situations requiring multi-component behaviour by modulating response selection processes. Participants We investigated n =18 (8 males, 10 females) right-handed (Edinburgh Handedness Inventory [28] , EHI=0.96±0.06) university students in their early twenties (23.8 years±1.8). All subjects had normal or corrected-to-normal vision, normal hearing capabilities and no history of neurological or psychiatric diseases, and conformed to current TMS safety criteria [29] , [30] . The study was approved by the ethics committee of the medical faculty of the Technische Universität Dresden. All subjects were thoroughly informed about the study protocol as well as possible risks, and gave written informed consent. The study complies with the Declaration of Helsinki. Experimental design The study consisted of four appointments. The first served to obtain the participants’ individual structural images and to assess the participants’ handedness, mental health and TMS safety criteria. In sessions two to four, we repeatedly recorded an electroencephalogram (EEG) while participants performed a stop–change task (see below). In each of the three sessions, a different TBS protocol was used. The protocols were either iTBS, cTBS or a shamTBS protocol (shamTBS). The protocol was applied immediately before the participants performed the stop–change task. Further details on the protocols are given below. The sequence of TBS protocols was counterbalanced across the n =18 subjects. Task We investigated the task goal processing strategy used during multi-component behaviour with the help of a stop–change paradigm previously employed by Mückschel et al. [1] The task was implemented using NBS Presentation software (Neurobehavioural Systems Inc.). Figure 1 , reproduced with permission from Stock et al. [4] , illustrates the task. Participants were seated in front of a 22-inch TFT screen at a distance of 1 m. For each session, the task consisted of six equally sized blocks. Each block consisted of 96 GO trials and 48 stop–change trials (SC trials) that were presented in a randomized order. Therefore, 864 trials were administered in the task, which took the participants ∼ 30 min to finish. Responses were given by pressing buttons on a custom response keypad (Cherry G86-63400, ZF Friedrichshafen AG) using the index and middle fingers of the right hand during the GO trials, and those of the left hand for the SC trials. Throughout each trial, a white rectangle of 20 × 96 mm was displayed on a black background in the centre of the screen. Within this rectangle, three horizontal reference lines (line thickness 1 mm, width 8 mm) separated four vertically aligned circles (diameter 8 mm). At 250 ms after the trial onset, one of the circles was filled white, thus becoming the GO target stimulus. In the GO condition (67% of all trials), the participant’s response was expected to indicate whether this target was located above or below the middle reference line. Responses were given by pressing the outer right key with the right middle finger (‘above’ judgment) or by pressing the inner right key with the right index finger (‘below’ judgment). All stimuli remained visible until the participant either responded or 2,500 ms had elapsed. When the RTs were longer than 1,000 ms, the German word ‘Schneller!’ (translating to ‘Faster!’) was presented above the box until the participant responded. The remaining 33% of trials were SC trials. The SC condition began with the presentation of a white GO stimulus. After a variable stop-signal delay (SSD), which was adjusted using a staircase procedure [3] , a STOP signal (a red rectangle replacing the previous white frame) was presented. This STOP signal remained on the screen until the end of the trial and requested the participant to try to inhibit the response to the GO stimulus. The SSD was initially set to 250 ms and was adapted to each participant’s performance by means of a staircase procedure to yield a 50% probability of successfully inhibited GO responses. In the case of a completely correct SC trial (no response to GO stimulus, no response prior to the CHANGE stimulus (explained below) in the SCD300 condition and a correct left-hand response to the CHANGE stimulus), the SSD of the following SC trial was adjusted by adding 50 ms to the SSD of the evaluated trial. In the case of an erroneous SC trial (if any of the above criteria were not met), the SSD was adjusted by subtracting 50 ms from the SSD of the evaluated trial. Limiting this procedure, the SSD values were set to not fall below a value of 50 ms and not to exceed a value of 1,000 ms. The staircase procedure was performed within the shamTBS condition, iTBS and cTBS conditions, respectively, that is, there was no criterion that was estimated, for example, in the shamTBS condition and then also used in the iTBS or cTBS condition. Because of this, the probability of successfully inhibiting the GO response was stable across TBS conditions. Irrespective of the stopping performance/inhibition, every stop signal was combined with one of the three possible CHANGE stimuli. The CHANGE stimulus was a 100-ms sine tone presented via headphones at 75 dB SPL and could be high (1,300 Hz), medium (900 Hz) or low (500 Hz) in pitch. The tone assigned a new reference line in relation to which the CHANGE stimulus (the previous white GO target circle on the screen) had to be judged. The high tone represented the highest of the three lines as the new reference, the medium tone represented the middle line and the low tone represented the lowest line (see Fig. 4 ). All three reference lines were used with equal frequency. The required CHANGE response had to be performed with the left hand. For this response, the RT (RT2) was measured. If the target was located above the newly assigned reference line, an outer left key press (left middle finger) was required; if the target circle was located below the newly assigned reference line, a left inner key press (left index finger) was required. In half of the SC trials, there was a SCD with a stimulus onset asynchrony (SOA) of 300 ms between the STOP and the CHANGE signals (SCD300 condition); in the other half of SC trials, the two stimuli were presented simultaneously (SOA of 0 ms, SCD0 condition). In the case of RT2s longer than 2000, ms, the German word ‘Schneller!’ (translating to ‘Faster!’) was presented above the box until the participant responded. During the inter-trial interval (fixed duration of 900 ms), a fixation cross was presented in the centre of the screen. Prior to the experiment, the participants performed an exercise until they began to understand the task. During this training procedure, subjects were trained before the experiment was started, that is, the participants were first familiarized with the GO response. Afterwards, they were familiarized with the pitches of the tones until they were able to classify the pitches with an accuracy of at least 90%. In a third step, they performed the task using a version in which the reference line indicated by the auditory stimuli was visually highlighted on the screen. After the participants performed this task version at an accuracy level of at least 90%, the main experiment was conducted. Estimating the strategy applied In the stop–change paradigm outlined above, three task goals were shown to be involved [3] during action cascading, that is, (i) responding to the GO signal, (ii) stopping with the stop signal and (iii) responding to the change signal. The strategy chosen to cascade these different task goals and actions (that therefore determined the efficiency of the process to activate these different task goals) was estimated using a mathematical model. As described above, the paradigm introduces two different SCD intervals. These intervals are important for the experimental logic and the estimation of the strategy applied due to capacity limits in the response selection processes. The SCD0 condition provides the participants with a ‘choice’ of how to process the STOP- and CHANGE-associated processes. Bottleneck models of response selection capacity limitations suggest that response selection can be performed serially (that is, one step is executed after another) or in parallel (that is, steps are processed in parallel so that there is a temporal overlap of processes [2] , [3] ). Because response selection depends on a restricted resource, the choice of which of these strategies to apply in STOP- and CHANGE-associated processes has consequences for the response selection processes and RTs on the CHANGE stimulus (RT2s). If participants choose to simultaneously process STOP- and CHANGE-associated task goals (that is, in parallel), RTs increase because these processes must share a limited capacity. However, in the SCD0 condition, the participants can also choose a strategy in which they process STOP- and CHANGE-associated task goals in a step-by-step (that is, serial) manner. If the participants choose a serial strategy, the STOP and CHANGE processes do not have to share a limited capacity when the STOP process is finished before the CHANGE process. This leads to shorter RT2s than the strategy in which STOP- and CHANGE-associated task goals are processed simultaneously. Critically, in the SCD300 condition, the SOA of 300 ms enforces a serial processing of the STOP- and CHANGE-related processes because the STOP process has finished when the CHANGE stimulus is presented 300 ms later. This condition therefore enables the estimation of which processing strategy has been used in the SCD0 condition. If a parallel processing strategy has been used in the SCD0 condition, RT2s are substantially longer in the SCD0 than in the SCD300 condition. If a serial processing strategy has been used in the SCD0 condition, the RT2s are comparable to those in the SCD300 condition. The ratio of RT2 differences in the SCD0 and SCD300 conditions therefore gives an estimate of the strategy used during action cascading [3] . This slope value was individually calculated for each participant. The value becomes steeper with increasing differences between RT2SCD0 and RT2SCD300. When the STOP process has not finished by the time the CHANGE process is initiated (parallel processing strategy), the slope value becomes larger, indicating that action cascading is less efficient. If the STOP process has finished (serial processing strategy), the slope approaches zero, which indicates that action cascading becomes more efficient [3] . Obtaining a mean slope value between 0 and −1 therefore suggests that some (but not all) of the CHANGE response processes were initiated prior to the termination of the inhibitory process stopping the GO response. Therefore, the slope of the SOA-RT2 function is flatter in the case of more efficient processing than in the case of the less efficient processing mode. MRI acquisition and TMS neuronavigation High-resolution three-dimensional T1-weighted anatomical brain images were acquired on a 3-Tesla HDxt whole-body MRI scanner (GE Signa) using an 8-channel head coil (BRAVO 8-channel brain) with magnetization-prepared gradient echo images (TR: 10.36 ms; TE: 4.2 ms; FA: 13°; 160 sagittal slices; matrix size, 512 × 512; FOV, 240 × 216 mm; 0.5 × 0.4 × 1.2 mm voxels). Structural images were prepared and neuronavigation was performed using the BrainVoyager TMS Neuronavigation System (BrainInnovation, Maastricht, The Netherlands) with established guidelines [31] . The rIFG’ target location was determined in a two-step process. First, group-based MNI coordinates of the rIFG were obtained from two previously reported studies. Verbruggen et al. [14] reported MNI coordinates of the ventral and dorsal regions of the rIFG and further showed that the ventral region is primarily involved in the updating of action plans rather than attentional processes. Further, Ness and Beste [32] reported MNI coordinates of the rIFG activated during an identical stop–change task executed during functional magnetic resonance imaging. Because we aimed to investigate the processes related to response selection, we calculated the mean rIFG MNI coordinates using the ventral rIFG MNI coordinates reported by Verbruggen et al. [14] and the rIFG MNI coordinates reported by Ness and Beste [32] . This initial target coordinate ([ x , y , z ]=[57, 21, 8]) was then converted to and marked on participants’ individual reconstructed right-brain hemispheres in Talairach space. Second, we optimized the individual fit with regard to anatomical landmarks to ensure the stimulation of the ventral rIFG. In a procedure that was analogous to Verbruggen et al. [14] ; that is, we identified the lateral sulcus, the inferior frontal sulcus and the precentral sulcus. The rIFG was directly anterior to the precentral sulcus; the vertical distance between the stimulation site and the lateral sulcus LS was ∼ 20% of the total distance between the lateral sulcus and the inferior frontal sulcus. This constituted the individualized final rIFG target location used during each of the participant’s TBS sessions. TMS neuronavigation was then performed in Talairach space using the BrainVoyager TMS Neuronavigation System. Continuous and intermittent TBS TMS was applied using a PowerMAG research 100 device (MAG & More GmbH, DE) equipped with a focal double coil (196 × 100 × 13.5 mm). To ensure stimulation accuracy, the participants were asked to place their heads on a custom-made chin rest. The resting motor threshold (RMT) was determined at the first laboratory session using a conventional protocol [33] , [34] with single TMS pulses applied to the primary motor cortex’s hand area (M1). The participants were familiarized with the TMS sensation at a low stimulation intensity of 40%. The intensity was then increased in steps of 10% of the device’s maximum stimulator output until the first motor evoked potential (MEP) was identified. Next, optimal M1 target location and coil positioning were adjusted to elicit a well-formed, peak-to-peak measured and reliable MEP. The RMT was assessed by sequentially increasing the intensity until five out of ten MEPs (peak-to-peak) of at least 50 μV were registered. In line with current safety standards [35] , we employed an inhibitory cTBS as well as a facilitatory iTBS protocol identical to that in Huang et al. [13] TBS consisted of bursts containing three pulses of 50 Hz at an intensity of 70% RMT repeated at 200-ms intervals (that is, at 5 Hz frequency). During each TBS session, 600 pulses were applied. For iTBS, a 2-s train of TBS was applied and repeated every 10 s for 40 repetitions. cTBS consisted of 40 s of continuous TBS. During TBS, the coil was positioned directly above and tangentially to the subject’s target point with the coil handle facing downwards. For sham stimulation, the coil was tilted away from the scalp in a 90° angle, and a rubber spacer was placed between the subject’s head and the coil (see Fig. 6a ). Accurate targeting was confirmed throughout the TBS stimulation using the neuronavigation system. EEG recording and analysis EEG activity was continuously recorded at a sampling rate of 5 kHz using TMS-compatible 60-channel EEG equipment (BrainAmp DC, BrainProducts). The recording reference was located at electrode site Fpz. Impedance levels were maintained below 5 kΩ. Offline EEG analysis was performed using BrainVision Analyzer 2 software (BrainProducts). For the EEG data analysis, the data were first down-sampled to 256 Hz and band-pass filtered (IIR: 0.5–20 Hz; at 48 db/oct each). Gross technical artefacts were removed during manual inspection. Recurring physiological artefacts, that is, eye blinks, saccades and pulse artefacts, were corrected using an independent component analysis (Infomax algorithm). Next, stop-stimulus-locked segments were formed. Automated artefact rejection procedures were applied (rejection criteria: maximum voltage step of more than 60 μV ms −1 , maximal value difference of 150 μV in a 250-ms interval, activity below 1 μV). Artefact rejection was followed by a current source density transformation, yielding a reference-free evaluation of the electrophysiological data and thus helping to identify the electrodes showing the strongest effects [36] . Baseline correction was conducted using the interval from −900 ms to −700 ms as the pre-stimulus baseline (that is, a baseline set prior to the occurrence of the GO stimulus). The electrodes used for the quantification of the P1, N1 and P3 ERPs were selected in a data-driven manner. On the basis of the scalp topography maps, the visual P1 and N1 were quantified at electrodes P7 and P8, respectively, (P1: 0 ms until 140 ms; N1: 150 until 250), the auditory P1 was quantified at electrodes C5 and C6, the auditory N1 was quantified at electrodes C5 and C6 (0 ms until 500 ms) and the P3 was quantified at electrode Cz (200 ms until 600 ms). The choice of electrode positions for data quantification was statistically validated as described in Mückschel et al. [1] All ERPs were quantified at the single-subject level. Latencies are given relative to the onset of the stop signal (time point 0), and amplitudes were quantified relative to the pre-stimulus baseline. Source localization analysis (sLORETA) Source localization was carried out to map the TBS-induced differences in the P3 ERP evoked in the SCD0 condition. Source localization was conducted using sLORETA [19] . sLORETA gives a single linear solution to the inverse problem based on extra-cranial measurements without a localization bias [19] , [37] , [38] . For sLORETA, the intracerebral volume is partitioned into 6.239 voxels at a 5-mm spatial resolution. The standardized current density of each voxel is calculated in a realistic head model [39] using the MNI152 template. In the present study, the voxel-based sLORETA images were compared across sessions (that is, cTBS versus shamTBS and iTBS versus shamTBS) using the sLORETA built-in voxel-wise randomization tests with 3,000 permutations based on nonparametric statistical mapping. Voxels with significant differences ( P <0.01, corrected for multiple comparisons) between groups were located in the MNI brain and Brodmann areas. Furthermore, coordinates in the MNI brain were determined using the sLORETA software ( www.unizh.ch/keyinst/NewLORETA/sLORETA/sLORETA.htm ). The results obtained using sLORETA have been shown to have high convergence with results from functional magnetic resonance imaging data. The algorithm provides reliable results without localization bias [38] . Statistical analysis The data were analysed using repeated measures ANOVAs with the within-subject factors ‘SCD interval’ (SCD0 versus 300), ‘condition’ (TBS protocols) and ‘electrode’ (wherever necessary). Post hoc tests were Bonferroni-corrected whenever necessary. All included variables were normally distributed as tested with Kolmogorov–Smirnov tests (all z <0.7; P >0.4). How to cite this article : Dippel, G. and Beste, C. A causal role of the right inferior frontal cortex in implementing strategies for multi-component behaviour. Nat. Commun. 6:6587 doi: 10.1038/ncomms7587 (2015).